The CDC13-STN1-TEN1 complex stimulates Pol α activity by promoting RNA priming and primase-to-polymerase switch Emerging evidence suggests that Cdc13-Stn1-Ten1 (CST), an RPA-like ssDNA-binding complex, may regulate primase-Pol α (PP) activity at telomeres constitutively, and at other genomic locations under conditions of replication stress. Here we examine the mechanisms of PP stimulation by CST using purified complexes derived from Candida glabrata . While CST does not enhance isolated DNA polymerase activity, it substantially augments both primase activity and primase-to-polymerase switching. CST also simultaneously shortens the RNA and lengthens the DNA in the chimeric products. Stn1, the most conserved subunit of CST, is alone capable of PP stimulation. Both the N-terminal OB fold and the C-terminal winged-helix domains of Stn1 can bind to the Pol12 subunit of the PP complex and stimulate PP activity. Our findings provide mechanistic insights on a well-conserved pathway of PP regulation that is critical for genome stability. Pol α, one of the three major replicative DNA polymerases in eukaryotes [1] , [2] , is distinguished from the other replicative polymerases in having a tightly associated primase activity [3] . The primase-Pol α (PP) complex consists of four subunits: Pol1, the DNA polymerase; Pol12, a ‘scaffold’ subunit that mediates interactions with regulatory factors [4] , [5] ; Pri1, the primase catalytic subunit; and Pri2, the large and non-catalytic primase subunit [6] , [7] . In chromosomal DNA replication, PP performs the task of the true initiator: it synthesizes a short RNA primer of ~7–10 nucleotides (nt) and extends it by an additional 10–20 dNMP before dissociating from the template/product duplex [8] , [9] . The 3′ terminus of the RNA–DNA chimera then serves as the primer for DNA synthesis by DNA polymerase ε and δ on the leading and lagging strands, respectively [10] . Although the DNA polymerase activity of Pol α can be assayed using synthetic template/primer substrates, prevailing evidence suggests a tight ‘communication’ between the primase and Pol α such that the latter preferentially extends RNA primers synthesized by the former subunit [9] . Telomeres, the special nucleoprotein structures located at the ends of linear eukaryotic chromosomes, are critical for chromosome stability; they protect the DNA termini from degradation, end-to-end fusion and other abnormal transactions [11] , [12] , [13] . Owing to the incomplete end-replication problem [14] , the maintenance of telomere DNA requires not only efficient semi-conservative DNA replication, but also terminal repeat addition. In most organisms, telomeric DNA consists of short repeats that are rich in G and C residues on the 3′- and 5′-end-bearing strands, respectively. These two complementary strands of telomeres, designated the G- and C-strands, are ‘extended’ sequentially by the telomerase and the PP complex; telomerase lengthens the G-strand through reverse transcription of an integral RNA template subunit [15] , [16] , [17] , whereas PP lengthens the C-strand by copying the extended G-tail [18] , [19] , [20] . The initial RNA–DNA chimera is presumably processed and ligated to the original 5′ end to yield the mature C-strand. Thus, the extension of telomeres is a multi-step process that entails the action of multiple enzymes, including PP. Because semi-conservative replication through telomeres also requires PP, this complex evidently participates in multiple telomere maintenance pathways and may thus be subjected to elaborate regulation at chromosome ends. Compelling evidence for special regulation of PP at telomeres came from analysis of the Cdc13-Stn1-Ten1 (CST) complex, a conserved G-strand-binding complex [21] , [22] , [23] . Initially discovered in the budding yeast Saccharomyces cerevisiae ( Sc ), the CST complex mediates critical functions in both telomere protection and maintenance. Mutations in subunits of the complex are often lethal, and hypomorphic alleles of CST genes were found to engender a wide variety of aberrations including telomere length alterations, telomere degradation and excessive recombination. Consistent with a role in telomere protection, the phenotypes of some CST mutants can be suppressed by checkpoint and nuclease mutations [24] , [25] . In support of the telomere maintenance function, CST is known to associate with both telomerase and PP subunits and is proposed to regulate the activity of both enzymes. Notably, the recent discovery and characterization of CST complexes in vertebrates suggest that PP regulation may be an especially well-conserved function of this complex [26] , [27] , [28] . In particular, the two largest subunits of the vertebrate complex (CTC1 (equivalent to fungal Cdc13) and STN1) were initially purified and analysed as Pol α-associated stimulatory factors (AAF-132 and AAF-44) [29] , [30] . Moreover, genetic depletion or disruption of vertebrate CST subunits does not cause immediate and generalized telomere de-capping, suggesting that the vertebrate complex plays a minor role in telomere protection [31] , [32] , [33] . Instead, loss of human or mouse CST subunits caused defects in telomere replication and C-strand fill-in synthesis, which are better explained by a function of CST in PP regulation at telomeres [31] , [32] , [33] , [34] , [35] . Depletion of vertebrate CST also impaired cellular recovery from replication stress, suggesting a non-telomeric function. Besides its multiplicity of functions, CST is notable for its resemblance to Replication protein A (RPA), the major single-stranded DNA (ssDNA)-binding complex in eukaryotes [36] , [37] . RPA, which mediates diverse functions in replication, recombination and repair, is also composed of three subunits (Rpa1, Rpa2 and Rpa3) [38] , and the two smaller subunits of the CST and RPA complexes manifest unmistakable structural and functional similarities [36] , [37] , [39] . Nevertheless, CST and RPA are clearly not redundant, and the distinctions between the two complexes are major topics of ongoing investigations. Notwithstanding the wealth of molecular genetic data on the role of CST in promoting DNA synthesis at telomeres and elsewhere, the biochemical mechanisms that undergird this regulation remain poorly understood. The physical basis for CST–PP interaction has not been elucidated. The precise molecular step(s) of the PP reaction cycle enhanced by the CST complex remains a subject of debate, with models favouring template binding, priming and DNA polymerization, all having been proposed [29] , [30] , [40] . Also unclear is the extent of evolutionary conservation between the vertebrate and fungal CST in regards to PP regulation. Studies of fungal CST mechanisms have been hampered by difficulties in isolating adequate quantities of the complex for detailed biochemical investigations. We recently overcame this obstacle by obtaining high levels of CST from Candida glabrata [41] , a pathogenic fungus that is evolutionarily close to S. cerevisiae . In this report, we explore the regulation of C. glabrata PP complex by CST and show for the first time that the PP stimulatory activity of CST is conserved in fungi. By characterizing the effect of CST on individual steps of the PP reaction cycle, we deduce that, while CST has no effect on the isolated DNA polymerase activity, it can substantially enhance the priming reaction and the primase-to-polymerase switch. We also home in on Stn1 as the CST subunit responsible for PP stimulation and show that this subunit makes multiple, functionally important contacts with the Pol12 subunit. Finally, we demonstrate that this pathway of PP regulation is extremely well conserved in evolution. Our findings establish a biochemical framework for interpreting the physiologic effects of CST. The PP complex catalyses the synthesis of RNA–DNA chimeras To investigate the regulation of PP by CST in vitro , we first isolated the two complexes encoded by C. glabrata . CST was obtained through recombinant co-expression and affinity purification from E. coli ( Supplementary Fig. 1a ) [41] , whereas PP through tagging of the Pri2 subunit and affinity purification from C. glabrata ( Supplementary Fig. 1b ). The PP complex can be further purified to near homogeneity by glycerol gradient fractionation ( Supplementary Fig. 1c ). The affinity-purified and glycerol gradient-purified PP behaved identically in all the polymerization assays used in the current study ( Supplementary Fig. 1d ). Before analysing the effect of CST, we characterized the synthesis of RNA–DNA chimeras by PP alone on poly-dT and two model G-tail substrates ( Fig. 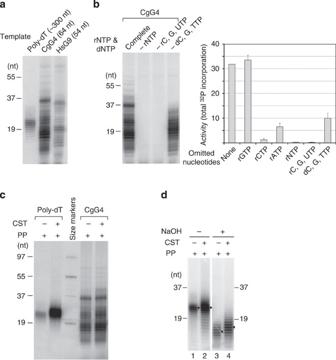Figure 1: Characterization of theC. glabrataPol α and the effect of CST on Pol α activity. (a)C. glabrataPP (2 nM) was subjected to coupled primase-polymerase assays using the indicated ssDNA templates (poly-dT at 300 nM, CgG4 and HsG9 at 1 μM). (b) PP (2 nM) was assayed using the CgG4 template and the indicated combinations of nucleotides. Total P32incorporation into the products was quantified from PhosphorImger scans and plotted. Data (averages±s.d.) are from three independent experiments. (c) The effect of CST (80 nM) on PP (1 nM) in the coupled primase-polymerase assays on poly-dT and CgG4 templates was analysed. (d) The PP reaction products generated in the absence and presence of CST were subjected to alkaline hydrolysis and analysed in a 13% acrylamide-TBE-urea gel. The peak product length for each sample is indicated by a black dot to the right. 1a ; Supplementary Table 1 ). Physiologic concentrations of ribonucleotides and deoxyribonucleotides (including P 32 -dATP) were used in the assays to mimic the in vivo condition [42] . Because the synthesis of detectable products required the action of both primase and DNA polymerase, this assay will be referred to as the coupled primase-polymerase assay. Labelled products that ranged in size from about 10 to 40 nt were generated in these reactions. The product size distribution was quite narrow for the poly-dT template, manifesting a sharp peak at ~20–25 nt. In comparison, the C-strand products were more heterogeneous in size such that short (10–20 nt) and long (30–40 nt) products were as well represented as the medium-sized products ( Fig. 1a ). As predicted for PP-mediated synthesis of C-strand RNA–DNA chimeras, product accumulation required the presence of both ribonucleotides and deoxyribonucleotides ( Fig. 1b ). Also consistent with the composition of the C. glabrata C-strand, omitting rCTP had a more detrimental effect than omitting other ribonucleotides on product synthesis. The different size distributions of the poly-dT and G-tail products indicate that the polymerization property of PP is sequence dependent, as noted in a recent study [43] . Figure 1: Characterization of the C. glabrata Pol α and the effect of CST on Pol α activity. ( a ) C. glabrata PP (2 nM) was subjected to coupled primase-polymerase assays using the indicated ssDNA templates (poly-dT at 300 nM, CgG4 and HsG9 at 1 μM). ( b ) PP (2 nM) was assayed using the CgG4 template and the indicated combinations of nucleotides. Total P 32 incorporation into the products was quantified from PhosphorImger scans and plotted. Data (averages±s.d.) are from three independent experiments. ( c ) The effect of CST (80 nM) on PP (1 nM) in the coupled primase-polymerase assays on poly-dT and CgG4 templates was analysed. ( d ) The PP reaction products generated in the absence and presence of CST were subjected to alkaline hydrolysis and analysed in a 13% acrylamide-TBE-urea gel. The peak product length for each sample is indicated by a black dot to the right. Full size image CST stimulates PP and alters the lengths of RNA and DNA Having detected PP activity on ssDNA templates, we next determined the effect of purified recombinant CST using this assay. In the standard coupled assay, CST stimulated the synthesis of RNA–DNA chimeras on poly-dT by ~fivefold and on the G-tail by approximately two- to threefold ( Fig. 1c ). Owing to the greater magnitude of stimulation, the detailed mechanism of PP stimulation by CST was characterized using primarily the poly-dT template. However, stimulation of PP activity on G-tail templates was also reproducibly observed, especially at low PP concentrations. Time course analysis indicates that for the poly-dT template the enhanced product accumulation in the presence of CST was due to an increase in the rate of synthesis ( Supplementary Fig. 2a ). The magnitude of stimulation was CST concentration dependent, reaching a maximum at ~100–150 nM ( Supplementary Fig. 2b ). The degree of stimulation was also affected by PP concentration, being highest at low-to-moderate levels of the polymerase in the presence of a fixed CST concentration ( Supplementary Fig. 2c,d ). Notably, these findings are consistent with early analyses of mammalian AAF [29] , [30] , suggesting that, despite the low level of sequence identity between the fungal and mammalian CST complexes (especially in regard to CTC1/Cdc13 and Ten1), the mechanism of PP regulation appears similar. CST not only stimulated product synthesis, but also caused a small but reproducible shift in the length distribution of the products; the centre of the product peak was longer by ~0.5–1.0 nt in the presence of CST compared with that found in its absence ( Fig. 1d , lanes 1 and 2; Supplementary Fig. 3a ). This alteration could be due to a change in the RNA or DNA length (or both) in the chimera. To distinguish between these possibilities, we subjected the products to alkaline hydrolysis, which completely removed the RNA portions from the chimeras. Remarkably, the centre of the ‘DNA only’ product peak was longer by ~1.5–2 nt when CST was included in the PP reaction ( Fig. 1d , lanes 3 and 4; Supplementary Fig. 3a ), implying that CST simultaneously shortened the RNA and lengthened the DNA synthesized by PP. We then used an alternative method to assess the lengths of the RNA primer, that is, by subjecting the chimeric products to DNase I treatment. This nuclease is known to cleave within the DNA portion of the chimera, leaving ~2–3 nt of labelled DNA attached to the RNA [8] . Interestingly, the most abundant cleavage product derived from the CST-plus reaction is ~1 nt shorter than that from the CST-minus reaction, again supporting the idea that CST shortened the RNA primer ( Supplementary Fig. 3b ). Our finding points to unexpectedly complex effects of CST on PP-mediated product synthesis. To assess the generality of the CST effects, we compared the distribution of products on G-tail templates. However, the heterogeneous nature of the C-strand products from the C. glabrata G-tail (CgG4) complicated the interpretation of results. We tested several alternative templates and found that one consisting of nine copies of the human G-strand repeat (HsG9) yielded regular and interpretable results ( Supplementary Fig. 3c ). On this template, several clusters of products that are ~6 nt apart can be detected in the absence of CST, presumably due to preferential initiation and termination of product synthesis at specific nucleotides within the repeat unit. Interestingly, the centre of the product peak within each cluster was also increased by about 1 nt in the presence of CST. Hence, the effect of CST on PP product lengths can be observed on both non-telomeric and telomeric templates. CST stimulates RNA priming and primase-to-polymerase switch A priori , the stimulatory effect of CST on total product synthesis can be due to an enhancement of the primase or DNA polymerase reaction, or the ‘coupling’ between the two active sites. To distinguish between these possibilities, we first analysed the effect of CST in separate primase and DNA polymerase reactions. For the primase-only assay, PP was incubated with poly-dT in the presence of labelled ATP as the sole nucleotide. Previous studies indicate that eukaryotic primase preferentially synthesizes unit-length primers (7–10 nt) or multiples thereof (that is, multiples of 7–10 nt) in the absence of dNTP. Indeed, we observed both unit-length primers and dimers in our assays ( Fig. 2a ). More interestingly, the effect of CST in this assay was ATP concentration dependent: CST stimulated primer synthesis by two- to threefold in 20 μM ATP, but had much less effect in 400 μM ATP ( Fig. 2a ). As a complementary test, we performed a standard primase assay, which combines primer synthesis (using unlabelled 3 mM ATP) with extension by Klenow (using labelled dATP) [2] . Because Klenow was included in excess, the dATP incorporation was proportional to the RNA primers produced in the reaction. Using this assay, we found little stimulation of primase activity by CST ( Fig. 2b ). Thus, CST preferentially enhances primase activity at low ATP concentrations. We then performed polymerase-only assays, for which we used ‘pre-primed’ Poly-dT/rA 10 template and dATP as the substrate ( Fig. 2c ). No enhancement of DNA synthesis was observed in the presence of CST, indicating that the complex does not stimulate the DNA polymerase activity. We reasoned that the DNA template/RNA primer generated by primase might behave differently from the synthetic Poly-dT/rA 10 substrate, and hence performed an alternative assay. In this assay, we first allowed PP to synthesize unlabelled oligo-rA using ATP as the sole nucleotide substrate. On completion of RNA synthesis, free ATP was removed from the reaction, and the resulting Poly-dT/oligo-rA mixture used as the substrate for DNA synthesis by PP in the absence or presence of CST ( Fig. 2d ). CST again had no effect on DNA synthesis, indicating that it does not stimulate ‘isolated’ DNA polymerase α activity. 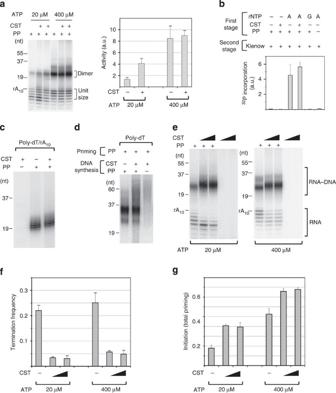Figure 2: CST promotes RNA priming and the primase-to-polymerase transition. (a) The primase activity of the PP complex (1 nM) was analysed at the indicated ATP concentrations in the absence or presence of CST (100 nM). Poly-dT was included at 300 nM, and P32-ATP was included at 12 and 2.4 μCi nmole−1for the 20 and 400 μM ATP reactions, respectively. Size standards in this and several other assays include both ssDNA (19, 37, 55 and 97 nt) and ssRNA (rA10). Results (averages±s.d.) from three independent assays were quantified and plotted. (b) The total32P incorporations for a series of coupled primase-Klenow assays are quantified and plotted. As controls, the priming step of the reactions was performed using no ribonucleotides or GTP only. Data (averages±s.d.) are from three independent sets of assays. (c) The DNA polymerase activity of PP (1 nM) was analysed in the absence or presence of CST (100 nM) using as substrates ‘pre-primed’ poly-dT/rA10(150 and 450 nM). (d) The DNA polymerase activity of PP (1 nM) was analysed in the absence or presence of CST (150 nM) using as substrates the poly-dT/oligo-rA synthesized by PP in a priming reaction. (e) The primase-to-polymerase switch efficiency of PP (2 nM) was analysed in the absence or presence of CST (100 and 200 nM) at the indicated ATP concentrations. P32-ATP was included at 24 and 1.2 μCi nmole−1for the 20 and 400 μM ATP reactions, respectively. (Because theKmof the primase for ribonucleotides is ~150 μM8, higher specific activity of P32-ATP is needed to generate robust signals in the 20 μM ATP reactions.) (f) The fractions of extendable RNA primers (that is, 7–10 nt long) that were not lengthened by the polymerase into RNA–DNA chimeras in assays such as those shown indwere quantified and plotted. Data (averages±s.d.) are from three independent sets of assays. (g) The total numbers of RNA and RNA–DNA products in assays such as those shown indwere calculated by summing the normalized intensities (normalized against the number of labelled rA in each product) and plotted. (For the RNA–DNA oligomer, we assume an average RNA length of 9.) Data (averages±s.d.) are from three independent sets of assays. Figure 2: CST promotes RNA priming and the primase-to-polymerase transition. ( a ) The primase activity of the PP complex (1 nM) was analysed at the indicated ATP concentrations in the absence or presence of CST (100 nM). Poly-dT was included at 300 nM, and P 32 -ATP was included at 12 and 2.4 μCi nmole −1 for the 20 and 400 μM ATP reactions, respectively. Size standards in this and several other assays include both ssDNA (19, 37, 55 and 97 nt) and ssRNA (rA 10 ). Results (averages±s.d.) from three independent assays were quantified and plotted. ( b ) The total 32 P incorporations for a series of coupled primase-Klenow assays are quantified and plotted. As controls, the priming step of the reactions was performed using no ribonucleotides or GTP only. Data (averages±s.d.) are from three independent sets of assays. ( c ) The DNA polymerase activity of PP (1 nM) was analysed in the absence or presence of CST (100 nM) using as substrates ‘pre-primed’ poly-dT/rA 10 (150 and 450 nM). ( d ) The DNA polymerase activity of PP (1 nM) was analysed in the absence or presence of CST (150 nM) using as substrates the poly-dT/oligo-rA synthesized by PP in a priming reaction. ( e ) The primase-to-polymerase switch efficiency of PP (2 nM) was analysed in the absence or presence of CST (100 and 200 nM) at the indicated ATP concentrations. P 32 -ATP was included at 24 and 1.2 μCi nmole −1 for the 20 and 400 μM ATP reactions, respectively. (Because the K m of the primase for ribonucleotides is ~150 μM [8] , higher specific activity of P 32 -ATP is needed to generate robust signals in the 20 μM ATP reactions.) ( f ) The fractions of extendable RNA primers (that is, 7–10 nt long) that were not lengthened by the polymerase into RNA–DNA chimeras in assays such as those shown in d were quantified and plotted. Data (averages±s.d.) are from three independent sets of assays. ( g ) The total numbers of RNA and RNA–DNA products in assays such as those shown in d were calculated by summing the normalized intensities (normalized against the number of labelled rA in each product) and plotted. (For the RNA–DNA oligomer, we assume an average RNA length of 9.) Data (averages±s.d.) are from three independent sets of assays. Full size image We then directly analysed the efficiency of primase-to-polymerase switch using labelled ATP and unlabelled dATP in the coupled assay. Strikingly, at both 20 and 400 μM ATP, CST increased the switch efficiency; the levels of unit-length primers were substantially reduced and the levels of RNA–DNA chimeras elevated ( Fig. 2e ). The characteristic increase in the length of the chimeric products was also observed. By quantifying the levels of RNA and RNA–DNA chimeras, we infer that CST reduced the termination frequency (that is, the fraction of 7-, 8-, 9- and 10-mer RNAs that were not lengthened to form RNA–DNA chimeras) from ~0.25 to ~0.05 ( Fig. 2f ). These findings provide direct support for the notion that CST stimulates DNA synthesis by raising the efficiency of the primase-to-polymerase switch. In addition, by quantifying the total number of RNA and RNA–DNA oligomers, we showed that CST stimulated RNA priming by approximately twofold at 20 μM ATP and by ~50% at 400 μM ATP ( Fig. 2g ). Thus, the overall increase in the level of RNA–DNA chimeras in the presence of CST is due to the combined effect of CST on the primase activity and the primase-to-polymerase switch. To examine further the mechanisms of stimulation, we performed a set of primer-capping assays, which are identical to switch assays, except that dATP is replaced by ddATP ( Supplementary Fig. 4 ) [44] . The capping assay allows RNA priming and switch to take place, but limits the extension of oligo-rA to a single deoxynucleotide. Because the oligo-rA-ddA products exhibit characteristic differences in mobility from the oligo-rA products, it is possible to assign the identity of the oligomers with high confidence, and thereby characterize the reactions in greater detail ( Supplementary Fig. 4a ). By comparing the product distributions in the unit-size primer range, we can clearly detect evidence for the stimulation of priming by CST in 20 μM ATP (compare traces 1 and 2, and 3 and 4 in Supplementary Fig. 4b ) and for stimulation of switch by CST in 400 μM ATP (compare traces 7 and 8 in Supplementary Fig. 4b ). Altogether, our collection of assays revealed multiple effects of the CST complex on different steps of nucleic acid synthesis by PP. The Stn1 subunit of CST is responsible for PP stimulation To determine the subunit(s) of the CST complex responsible for PP stimulation, we prepared and tested isolated subunits. Each subunit was expressed in Escherichia coli , purified by affinity chromatography ( Supplementary Fig. 1a ) and found to be free of contaminating polymerase activity. Notably, neither Cdc13 nor Ten1 was capable of stimulating PP. Because we had previously shown that recombinant Cdc13 alone is active in DNA binding, its inability to stimulate PP cannot be attributed to gross misfolding [41] . In contrast to Cdc13 and Ten1, Stn1 alone was nearly active as the intact CST complex in PP stimulation ( Fig. 3a ). The effect of Stn1 can be observed on both the Poly-dT and C. glabrata G-tail templates ( Fig. 3a , left and right panels). Stn1 contains an amino-terminal oligonucleotide/oligosaccharide-binding (OB) fold domain that is implicated in DNA binding and a carboxy-terminal duplicated winged-helix domain that is proposed to contact other proteins [36] , [37] , [39] , [41] . We purified these two domains separately ( Supplementary Fig. 1a ) and found that each was competent in PP stimulation ( Fig. 3b ). All the Stn1 variants (that is, full length, N terminus and C terminus) caused the characteristic lengthening of products described earlier for the intact CST complex, suggesting that their mechanisms of stimulation are likely to be similar. Titration of CST and Stn1 variants in the Poly-dT assays indicates that CST, Stn1 and Stn1N have comparable activities, while Stn1C is somewhat less active in PP stimulation ( Fig. 3c,d ). Thus, the PP-regulatory function of CST appears to reside largely in the Stn1 subunit, which possesses at least two determinants for promoting PP activity. 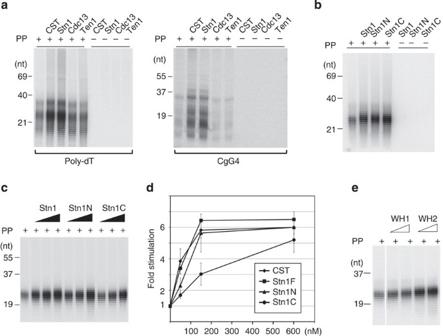Figure 3: Stimulation of PP activity by CST, Stn1 and Stn1 variants. (a; Left) The effects of CST complex and individual subunits (450 nM) on PP activity (2 nM) were analysed in the coupled primase-polymerase assays using the poly-dT template. (Right) The effects of CST complex and individual subunits (450 nM) on PP activity (2 nM) were analysed in the coupled primase-polymerase assays using the CgG4 template. (b) The effects of full-length Stn1 and the N- and C terminus of Stn1 (1 μM) on PP (2 nM) activity were analysed in the coupled primase-polymerase assays using poly-dT template. (c) PP (1 nM) activity was assayed using poly-dT and varying concentrations (75, 150 and 600 nM) of Stn1, Stn1N and Stn1C. (d) The stimulatory effects (averages±s.d.) of varying concentrations of CST, Stn1, Stn1N and Stn1C from three independent experiments were quantified and plotted. (e) The stimulatory effects of WH1 and WH2 motifs of Stn1C (at 100 and 300 nM concentrations) were analysed in the coupled primase-polymerase assays using the poly-dT template. The assays were from the same gel with several irrelevant lanes cropped out. Figure 3: Stimulation of PP activity by CST, Stn1 and Stn1 variants. ( a ; Left) The effects of CST complex and individual subunits (450 nM) on PP activity (2 nM) were analysed in the coupled primase-polymerase assays using the poly-dT template. (Right) The effects of CST complex and individual subunits (450 nM) on PP activity (2 nM) were analysed in the coupled primase-polymerase assays using the CgG4 template. ( b ) The effects of full-length Stn1 and the N- and C terminus of Stn1 (1 μM) on PP (2 nM) activity were analysed in the coupled primase-polymerase assays using poly-dT template. ( c ) PP (1 nM) activity was assayed using poly-dT and varying concentrations (75, 150 and 600 nM) of Stn1, Stn1N and Stn1C. ( d ) The stimulatory effects (averages±s.d.) of varying concentrations of CST, Stn1, Stn1N and Stn1C from three independent experiments were quantified and plotted. ( e ) The stimulatory effects of WH1 and WH2 motifs of Stn1C (at 100 and 300 nM concentrations) were analysed in the coupled primase-polymerase assays using the poly-dT template. The assays were from the same gel with several irrelevant lanes cropped out. Full size image Stn1 makes multiple contacts with Pol12 The complex effect of CST and Stn1 on PP products suggests allosteric control that could be mediated by protein–protein interactions between subunits of the two complexes. The putative interaction between CST and PP was confirmed using a glutathione S-transferase (GST) pull-down assay. Purified CST complex was immobilized on glutathione-Sepharose through the GST tag on Ten1. Whole-cell extracts from the C. glabrata strain carrying FLAG 3 -tagged Pri2 were incubated with the CST-containing beads, and CST-associated proteins in pull-down samples analysed for polymerase activity as well as Pri2-FLAG 3 protein. As predicted, the CST pull-down samples contained higher levels of polymerase activity as well as Pri2-FLAG 3 , indicating that the two complexes can physically associate with each other ( Supplementary Fig. 5 ). Previous analysis points to two possible contacts between CST and PP: one between Cdc13 and Pol1 and the other between Stn1 and Pol12 (refs 19 , 45 , 46 ). That Stn1 alone but not Cdc13 is able to stimulate PP suggests that the latter interaction may be functionally more important. We therefore examined the physical interaction between Stn1 and Pol12 using a co-expression/affinity purification assay. The two proteins were expressed separately or together in E. coli as His 6 -SUMO and GST-FLAG fusion proteins, respectively. Extracts were prepared and subjected to affinity purification to assess complex formation. As hypothesized, His 6 -SUMO-Stn1 and GST-FLAG-Pol12 remained stably associated with each other following both Ni-NTA and anti-FLAG affinity chromatography ( Fig. 4a ). Moreover, the two polypeptides are present at a 1:1 ratio, suggesting a 1:1 stoichiometry. Surprisingly, when Stn1 and Pol12 were first separately purified, and then subjected to anti-FLAG or glutathione pull-down assays, little interaction was detected between the two proteins. This observation suggested that one of the proteins may adopt an unproductive conformation when it is expressed in the absence of the other. Because Stn1 alone is active in PP stimulation, we suspect that isolated Pol12 may adopt an aberrant conformation. Indeed, an existing crystal structure of the Sc Pol1-Pol12 complex revealed extensive contacts between Pol12 and the C terminus of Pol1 (ref. 47 ), suggesting that Pol1 may influence Pol12 conformation. We then tested the N- and C-terminal domains of Stn1 and found that each domain can independently bind Pol12 ( Fig. 4b ). Thus, the ability of both the N- and C terminus of Stn1 to stimulate PP activity correlates with their binding to Pol12. 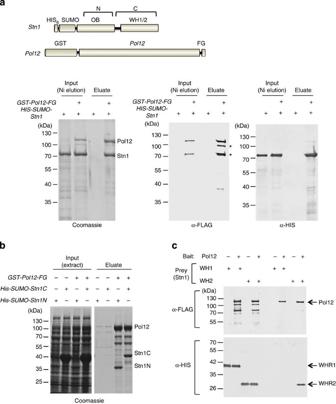Figure 4: The physical interaction between Stn1 and Pol12. (a) A schematic depiction of the fusion tags used for the co-expression/pull-down assays is shown at the top. Fractions derived from Ni-NTA purification of extracts containing Stn1 alone or Stn1 and Pol12 were subjected to anti-FLAG (M2) affinity purification. The input and purified fractions were subjected to SDS–polyacrylamide gel electrophoresis, Coomassie staining and western blot analysis using the indicated antibodies. Two proteolytic fragments of Pol12 detected by anti-FLAG western blot are indicated by asterisks. (b) Extracts from strains expressing Stn1 domains alone or in combination with Pol12 were subjected to M2 affinity purification, and the input and purified fractions analysed by SDS–PAGE and Coomassie staining. (c) Extracts from strains expressing Stn1C WH1 or WH2 motifs alone or in combination with Pol12 were subjected to GST affinity purification, and the input and purified fractions analysed by western blot. Pol12 was detected by anti-FLAG, whereas WH1 and WH2 by anti-HIS antibodies. Figure 4: The physical interaction between Stn1 and Pol12. ( a ) A schematic depiction of the fusion tags used for the co-expression/pull-down assays is shown at the top. Fractions derived from Ni-NTA purification of extracts containing Stn1 alone or Stn1 and Pol12 were subjected to anti-FLAG (M2) affinity purification. The input and purified fractions were subjected to SDS–polyacrylamide gel electrophoresis, Coomassie staining and western blot analysis using the indicated antibodies. Two proteolytic fragments of Pol12 detected by anti-FLAG western blot are indicated by asterisks. ( b ) Extracts from strains expressing Stn1 domains alone or in combination with Pol12 were subjected to M2 affinity purification, and the input and purified fractions analysed by SDS–PAGE and Coomassie staining. ( c ) Extracts from strains expressing Stn1C WH1 or WH2 motifs alone or in combination with Pol12 were subjected to GST affinity purification, and the input and purified fractions analysed by western blot. Pol12 was detected by anti-FLAG, whereas WH1 and WH2 by anti-HIS antibodies. Full size image To characterize the functional significance of Stn1–Pol12 interaction, we further dissected the C-terminal winged-helix domain of Stn1, which contains two winged-helix repeats, named WH1 and WH2. Each repeat was expressed and purified as a His 6 -SUMO fusion protein and then tested for PP stimulatory activity on the poly-dT template. Only WH2 showed significant stimulatory activity, implying that this repeat is responsible for the stimulatory function of Stn1C ( Fig. 3e ). Indeed, only WH2 showed detectable binding to Pol12 in the co-expression/pull-down assay, suggesting that the physical interaction is necessary for Stn1-mediated PP stimulation ( Fig. 4c ). We also attempted to identify point mutations in Stn1C that disrupt the Stn1–Pol12 interaction. The mutations examined are clustered near the central β-sheet of the winged-helix repeats, which is thought to be the main protein-binding surface in this motif [48] . Several of the alleles correspond to S. cerevisiae alleles that were previously shown to cause telomere lengthening [36] . Altogether, we generated and analysed five Stn1C mutant alleles, two in the first and three in the second winged-helix repeat ( Supplementary Table 2 ; Supplementary Fig. 6a ). Interestingly, none of the substitution mutants lost its association with Pol12, even though most mutant alleles were expressed at lower levels than wild-type Stn1C, possibly due to structural perturbations ( Supplementary Fig. 6b ). Consistent with the binding results, all of the point mutants retained stimulatory function in PP activity assays ( Supplementary Fig. 6c ). Thus, The WH2 motif of Stn1C may use a novel, non-β-strand surface to mediate Pol12 binding and PP stimulation. In addition, the telomere-lengthening effect of comparable Sc STN1 mutations was probably not due to altered binding to Pol12. Conservation of PP regulation by Stn1 in fungi and humans Even though mammalian CST is known to bind and stimulate mammalian PP, the mechanistic basis of this regulation is largely undefined. To determine whether the mechanisms we defined in fungi are applicable to other organisms, we examined the activities of purified human PP ( Hs PP) and human STN1 ( Hs STN1) using the same assays. In the standard coupled assays on the poly-dT template, Hs PP generated chimeric products that are slightly longer than those of Cg PP, but otherwise displayed similar properties with respect to template and nucleotide utilization ( Fig. 5a , lanes 1 and 4). In general agreement with the fungal studies, hs STN1 alone stimulated product synthesis by hs PP and increased the lengths of the RNA–DNA chimera slightly ( Fig. 5a , lanes 1 and 2). Likewise, in the primase-to-polymerase switch assays, hs STN1 increased the total number of RNA and RNA–DNA oligomers (by ~70%) and reduced the fraction of the RNA primers that terminated at the priming stage (by ~30%; Fig. 5b ). (Note that, while the levels of unextended RNA oligomers were similar in lanes 1, 2 and 3, the higher levels of total reaction products in lanes 2 and 3 indicate that the fractions of unextended RNA primers were lower for these two reactions.) Remarkably, despite the very low level of sequence similarity between Cg Stn1 and Human STN1 ( Hs STN1; ~17% identity and 33% similarity), both proteins displayed substantial stimulatory activities on the heterologous PP complex ( Fig. 5a ). In a side-by-side comparison of the two proteins in Poly-dT assays over a range of concentrations, Hs STN1 is only about twofold less active than Cg Stn1 in stimulating Cg PP ( Supplementary Fig. 6d ). 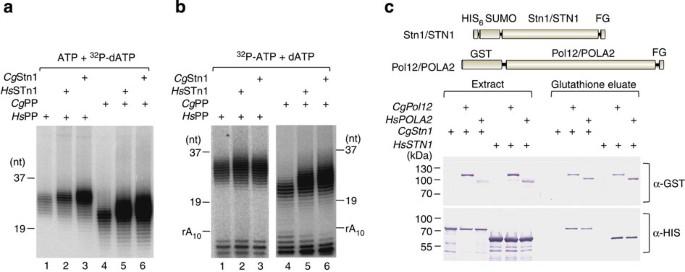Figure 5: The intra-species and inter-species binding and stimulatory activities ofC. glabrataand human Stn1. (a)HsPP andCgPP were analysed in the absence or presence ofHsSTN1 orCgStn1 using the poly-dT template, unlabelled ATP and labelled dATP. (b)HsPP andCgPP were analysed in the absence or presence ofHsSTN1 orCgStn1 using the poly-dT template, labelled ATP and unlabelled dATP. (c) Extracts from strains expressing the indicated combinations of Pol12 and Stn1 were subjected to GST affinity purification, and the extracts and purified fractions analysed by western blot using anti-HIS and anti-GST antibodies. Figure 5: The intra-species and inter-species binding and stimulatory activities of C. glabrata and human Stn1. ( a ) Hs PP and Cg PP were analysed in the absence or presence of Hs STN1 or Cg Stn1 using the poly-dT template, unlabelled ATP and labelled dATP. ( b ) Hs PP and Cg PP were analysed in the absence or presence of Hs STN1 or Cg Stn1 using the poly-dT template, labelled ATP and unlabelled dATP. ( c ) Extracts from strains expressing the indicated combinations of Pol12 and Stn1 were subjected to GST affinity purification, and the extracts and purified fractions analysed by western blot using anti-HIS and anti-GST antibodies. Full size image The ‘cross-species’ stimulation of PP by Stn1 suggests that the protein interface between Pol12 and Stn1 may be quite similar in humans and C. glabrata . To test this possibility, we examined all the potential pair-wise interactions between the Pol12 and Stn1 orthologues from C. glabrata and humans using the co-expression/affinity purification assay described in the previous section. Consistent with a high degree of conservation of the Stn1–Pol12 interface, we observed co-purification between all the intra-species and inter-species protein pairs on glutathione-Sepharose ( Fig. 5c ). We surmise that the relevant features of the Stn1–Pol12 interaction have been preserved between fungi and mammals not withstanding one billion years of evolution. The chief significance of the current report resides in the demonstrations that the fungal CST complex stimulates PP activity in vitro , that this regulation is due to an enhancement of both RNA priming and the primase-to-polymerase switch, that Stn1–Pol12 interaction provides the physical basis for this regulation and that this regulatory mechanism is well conserved in evolution. The implications for these findings are discussed below. Seminal studies on the priming and switch reactions, as well as recent structural analysis of the holoenzyme offer a framework for interpreting the current results [8] , [9] , [44] . The early experiments indicate that (i) only primers of sufficient lengths (seven nucleotides or longer) can be utilized by the DNA polymerase and (ii) the efficiency of the primase-to-polymerase switch is highly dependent on temperature, template concentration and deoxynucleotide concentration. In general, conditions that favour the stability and formation of RNA–DNA hybrid (for example, low temperature and high template concentration) or DNA synthesis (for example, high deoxynucleotide concentration) appear to enhance the switch efficiency [8] . The recent structural analysis of the architecture of the PP complex provides additional clues to the ‘switch’ process. On the basis of cryo-electron microscopy image reconstruction, the holoenzyme adopts a dumbbell configuration with two mobile lobes [44] . One lobe is occupied by the catalytic domain of Pol1 and the other by Pol12, Pri1, Pri2 and the C-terminal domain of Pol1, respectively. This model suggests plausible means by which Stn1 regulates priming and the switch reaction. For example, Pol12, on binding Stn1, is well positioned to regulate primase activity because of their close physical proximity. In addition, the large distance between the centres of the two PP lobes (the presumed active sites of the enzymes) implies that a coordinated conformational change may be required for the handoff reaction [44] . One possible consequence of Stn1–Pol12 interaction may hence be a conformational change in PP that brings the two lobes closer together to enhance the coordination between the active sites. More efficient transfer of the DNA–RNA hybrid from the primase-to-polymerase active site may also enable a greater fraction of short RNA primers (which are less-efficient substrates for the DNA polymerase) to be extended into chimeric products, resulting in a shortening of the average length of the RNA in the chimera. Structural and single-molecule analyses will likely be necessary to achieve understanding of the physical basis of the complex regulatory effects of CST on PP. The modulation of the primase-to-polymerase switch represents an unprecedented means for regulating PP activity. Our finding raises the possibility that other factors may regulate PP in a similar manner. In particular, the paralogous RPA complex has been reported to stimulate the DNA polymerase activity and processivity of Pol α [49] . However, the stimulatory activity of RPA was attributed to Rpa1 rather than the Stn1 paralogue Rpa2. Because the substrates and assays used in the RPA study are different from those in the current report, the potential role of Rpa2 in PP stimulation warrants further investigation. In this regard, we note that Rpa2 also possesses an N-terminal OB fold and a C-terminal winged-helix domain (albeit just one iteration of the winged-helix motif). The discovery of the PP stimulatory activity of the C. glabrata CST complex adds to the growing evidence for functional conservation between vertebrate and fungal CST, previously thought to be limited because of poor sequence conservations between subunits of the complexes and the very different routes of discovery. As noted before, while the fungal CST complex was initially characterized as a telomere-capping complex, the vertebrate factors were initially purified owing to their Pol α stimulatory activity. Even though studies to date have not revealed a direct telomere-protective function for vertebrate CST, the current report leaves little doubt that the fungal complex stimulates PP. Thus, PP regulation appears to be a more ancient and conserved function of CST, whereas telomere capping a more recent and specific acquisition of the fungal complex. Moreover, the mechanisms of PP enhancement appear to be similar if not identical between the fungal and vertebrate complexes, as evidenced by the ability of both Hs STN1 and Cg Stn1 to stimulate priming and the primase-to-polymerase switch. Indeed, the ability of fungal and human Stn1 to bind heterologous Pol12 and stimulate heterologous PP indicates that the Stn1–Pol12 interface has been retained through one billion years of evolution. The regulatory mechanism we uncovered is likely to extend to non-fungal and non-vertebrate organisms because most Stn1s in these organisms also contain an N-terminal OB fold and a C-terminal duplicated winged-helix domain. Thus, they have the potential of making multiple contacts to Pol12 to stimulate PP. An interesting case is presented by the plant Stn1 orthologues, which are unusually small and lack the C-terminal winged-helix domain [50] . Nevertheless, because the OB fold domain of Cg Stn1 alone exhibits a PP stimulatory activity, this function could very well be conserved in the plant homologues as well. Two intriguing notions concerning the regulation of DNA replication in vivo can be proposed based on previous findings and the current observations. The first relates to the control of dormant origins. As noted before, CST is implicated in replication at telomeres constitutively and elsewhere under conditions of replication stress [31] , [32] , [33] , [34] , [35] . Interestingly, at least in the context of hydroxyurea-mediated replication stress, CST appears to promote the firing of dormant origins, but not fork restart [32] . Our data suggest that CST may regulate PP both at the priming and the primase-to-polymerase switch steps, implying that these could be the rate-limiting steps for dormant origin firing in vivo . The second notion concerns the role of CST and Pol α in checkpoint regulation. Pol α has long been known to play a role in S-phase checkpoint activation, but the underlying mechanisms are poorly understood [51] , [52] , [53] . A recent report demonstrates that overexpression of Stn1C in S. cerevisiae renders the cells highly sensitive to HU by blocking aspects of S-phase checkpoint [54] . Curiously, the signalling cascade that leads to Rad53 phosphorylation remains active, but origin firing becomes resistant to the suppressive checkpoint signals. Moreover, the sensitivity of Stn1C-overproducing cells to HU appears to require Stn1–Pol12 interaction. Our observation that Stn1C can stimulate priming and the primase-to-polymerase transition suggests that these steps may be under S-phase checkpoint control and that misregulation of these steps by pathologic concentrations of Stn1C may overcome checkpoint inhibition of DNA replication. Strains and plasmids The C. glabrata strain BG14 ( ura3 ::Tn903 G418 R , a gift from Brendan Cormack, Johns Hopkins University) was used for the introduction of the tagged PRI2 gene [55] . For construction of FLAG 3 -tagged PRI2 , the full PRI2 open reading frames (ORF) with ~500 base pair of 5′ and 3′ flanking sequences was amplified by PCR and inserted between the XhoI and XbaI sites of the pGRB2.0 plasmid. The 3′ end of the PRI2 ORF was modified by Quikchange mutagenesis, resulting in the introduction of consecutive AvrII and BspEI restriction sites. A double-stranded oligo carrying the FLAG 3 tag was then inserted between the two sites to yield pGRB2.0-PRI2-FG. The plasmid was transformed into BG14 , and the resulting strain used for PP purification. Purification of Pol α, CST, Cdc13, Stn1 and truncation variants The PP complex was purified from C. glabrata as follows: the BG14 strain carrying pGRB2.0-PRI2-FG was grown in selective medium overnight until saturation. A suitable volume of saturated culture was used to inoculate 3-l YPD (1% yeast extract, 2% peptone, 2% glucose) such that the initial OD 600 (optical density) was ~0.5. The culture was grown to an OD 600 of 2.5, harvested and re-suspend in Buffer TMG (10 mM Tris HCl, pH 8.0, 1.2 mM MgCl 2 , 0.1 mM EDTA, 0.1 mM EGTA, 200 mM Na-acetate, 10% glycerol) at a ratio of 1 ml buffer per gram wet weight. The cells were lyzed by vortexing the suspension with an equal volume of glassbeads for a total of ~20 min (2 min pulses interspersed with 3 min cooling in an ice-water bath). S100 supernatant was prepared by centrifuging the lysate in T-875 rotor (Sorvall) at 32,000 r.p.m. for 1 h. Extracts were subjected to M2 affinity purification as follows. The extracts were adjusted to the 2.5 mM MgCl 2 , 1 mM dithiothreitol (DTT), 0.1% NP-40 and incubated with 1/80 vol of M2-agarose resin at 4 °C on a rotator for 4 h. The resin was then washed five times with the FLAG(150) buffer (50 mM Tris.HCl, pH 7.5, 250 mM NaCl, 10% glycerol, 0.1% NP-40, 2.5 mM MgCl 2 , 1 mM DTT) and eluted with FLAG(150) buffer containing 0.2 mg ml −1 FLAG 3 peptide. For some assays, the M2-purified PP complex was further purified on a 5-ml 15–30% glycerol gradient in buffer G (50 mM Tris HCl, pH 7.5, 150 mM NaCl, 2 mM DTT, 0.1% Triton X-100). The gradient was centrifuged at 42,000 r.p.m. for 15 h using a Sorvall AH-650 rotor. Twenty-five fractions were collected and assayed for polymerase activity and Pri2-FLAG 3 levels. The human PP complex was prepared by mixing equal molar concentrations of purified PRI1-PRI2 (from E. coli ) and purified POL1-POL12 complexes (from insect cells) as previously described [56] . The CST complex was purified from E. coli that carries expression plasmids for all three subunits as previously described [41] . Cdc13, Stn1, Stn1N, Stn1C, WH1, WH2 and human STN1were each purified as His 6 -SUMO-FLAG fusion proteins by sequential affinity chromatography as follows. The relevant ORFs with a C-terminal FLAG tag were generated by PCR and cloned downstream of the T7 promoter and the His 6 -SUMO tag in the pSMT3 vector. The expression plasmid was introduced into the BL21(DE3) codon plus strain and the proteins purified through Ni-NTA and M2 agarose. Ten1 was purified as a GST fusion protein using the pGEX-6P1 vector (GE Healthcare), the BL21(DE3) codon plus strain and glutathione-Sepharose as previously described [41] . The concentrations of the proteins were all estimated by comparing their Coomassie staining intensities with a standard curve of specified quantities of bovine serum albumin. In the case of PP, the concentration was calculated based on the staining intensity of the Pol1 subunit. PP activity assays and product analysis Unless otherwise indicated, the coupled primase-polymerase assays were performed in 20 μl volume containing 40 mM Tris HCl, pH 7.6, 30 mM potassium acetate, 13 mM Mg acetate, 5 mM DTT, 0.05 mM EDTA, 5% glycerol, 0.1 mg ml −1 bovine serum albumin, ~1–2 nM Pol α, ~40–120 nM CST (or CST subunits), 3 mM ATP, 0.5 mM CTP, 0.7 mM GTP, 1.7 mM UTP, 16 μM dATP, 14 μM dCTP, 12 μM dGTP, 30 μM dTTP and various labelled nucleotides or deoxynucleotides. In the standard coupled primase-polymerase assay, P 32 -dATP (5 μCi nmole −1 ) was included. The concentration of poly-dT template DNA (~300 nt, Midland Certified Reagent Company) was 300 nM, and that of the CgG4 (64 nt) and HsG9 (54 nt) template 1 μM. In some Poly-dT assays, only ATP and dATP were included. After incubation at 32 °C for 60–90 min, reactions were treated with 100 μl STOP solution (20 mM Tris HCl, pH 8.0, 20 mM EDTA) and 100 μl proteinase K solution (10 mM Tris HCl, pH 8.0, 0.5% SDS, 0.15 mg ml −1 proteinase K) and incubated at the same temperature for 30 min. For the primase-to-polymerase switch assays that detect simultaneously RNA and RNA–DNA oligomers, we replaced P 32 -dATP with 16 μM cold dATP and cold ATP with P 32 -ATP. The specific activities of P 32 -ATP used are indicated in the relevant figure legends. The primase-capping assays were identical to the switch assay, except that cold dATP was replaced by ddATP. For the ‘primase only’ assays, labelled ATP was used as the sole nucleotide substrate. For the Klenow-based primase assays, the primase reaction was performed with or without CST using 3 mM unlabelled ATP as the only nucleotide. The DNA template/RNA primer products were then recovered and subjected to Klenow extension in the presence of labelled dATP [2] . To test just the DNA polymerase activity, we used poly-dT/rA 10 (150 nM poly-dT and 450 nM rA 10 ) as the pre-primed substrate and labelled dATP as the sole nucleotide. For an alternative DNA polymerase assay, the priming reaction was performed in the absence of CST using 3 mM unlabelled ATP as the only nucleotide. On completion of the primase reaction, the mixture was adjusted to 50 μl containing 25 mM EDTA, 0.25% SDS and 0.2 mg ml −1 proteinase K. After 30 min incubation at 32 °C, the mixture was extracted once with phenol/chloroform/isoamyl alcohol and then passed through a Centri-Spin 20 column (Princeton Separations) to remove free ATP. The template and oligo-rA primer were then recovered by ethanol precipitation and used as substrates for PP and CST in assays that use labelled dATP as the sole nucleotide. To remove the RNA portions of the RNA–DNA chimeras, the products were incubated in 100 μl of 0.3% SDS and 20 mM EDTA at 55 °C for 10 min, followed by the addition of 15 μl 2.5 M NaOH and a further 2 h incubation at 55 °C. The mixture was then neutralized by adding 25 μl 2 M acetic acid, and the DNA recovered by ethanol precipitation [57] . For DNase I treatment, the reaction products from the coupled assays were incubated with 1 U DNase I at 37 °C for 2 h followed by ethanol precipitation. Pilot experiments indicate that longer incubation or additional DNase I did not result in further degradation of the chimera. For electrophoretic analysis, the products from the various assays were recovered by ethanol precipitation in the presence of 2.5 M ammonium acetate, 15 μg ml −1 glycogen and 15 μg ml −1 transfer RNA. The samples were dissolved in 90% formamide, 20 mM EDTA, 1 mg ml −1 xylene cyanol and 1 mg ml −1 bromophenol blue, boiled for 5 min and then applied to a denaturing polyacrylamide gel. Three different gel recipes were used depending on the nature of the experiments. For standard poly-dT assays, products were analysed in 13% acrylamide/7 M urea/1 × TBE gels. For assays designed to characterize short RNA oligomers, products were analysed in 18% acrylamide/7 M urea/1 × TBE gels [8] . For assays with G-tail templates, products were analysed in 10% acrylamide/7 M urea/36% formamide/1 × TBE gels. The high formamide concentration was needed to fully denature the extremely GC-rich template/product duplexes. Analysis of Stn1–Pol12 interaction The co-expression/pull-down assays were performed as follows [58] . The DNAs encoding the various Stn1 and Pol12 fragments (see Supplementary Table S2 for the amino acids included in each expression construct) were amplified by PCR and cloned into the pSMT3 vector [59] and the pGEX6P-1vector (GE Healthcare) to enable their expression as HIS 6 -SUMO and GST-FLAG fusion proteins, respectively. Each HIS 6 -SUMO fusion protein was expressed alone or co-expressed with a GST-FLAG fusion protein in E. coli BL21 (DE3). The growth and induction protocols as well as the extract preparation procedures were as previously described [60] . For Anti-FLAG pull-down assays, ~500 μl of 10 mg ml −1 extract was incubated with 20 μl of M2-agarose beads (Sigma) in the FLAG(250) buffer (50 mM Tris HCl, pH 7.5, 250 mM NaCl, 10% glycerol, 0.1% NP-40, 2.5 mM MgCl 2 , 1 mM DTT). Following incubation with constant mixing on a rotator at 4 °C for 2 h, the beads were washed five times with 0.5 ml of the FLAG(150) buffer, and then the M2-bound proteins eluted with 60 μl FLAG(150) containing 0.2 mg ml −1 3 × FLAG peptide. The eluates were analysed by SDS-polyacrylamide gel electrophoresis, followed by staining with Coomassie Brilliant Blue R-250 or western blotting. The GST pull-down assays were carried out using glutathione-Sepharose (GE Healthcare). The binding and washing buffers were identical to those of the M2 pull-down assays, and the elution buffer consists of FLAG(150) supplemented with 15 mM reduced glutathione. How to cite this article: Lue, N. F. et al . The CDC13-STN1-TEN1 complex stimulates Pol α activity by promoting RNA priming and primase-to-polymerase switch. Nat. Commun. 5:5762 doi: 10.1038/ncomms6762 (2014).